Smurf2 suppresses B-cell proliferation and lymphomagenesis by mediating ubiquitination and degradation of YY1 About half of patients with diffuse large B-cell lymphoma (DLBCL) do not respond to or relapse soon after the standard chemotherapy, indicating a critical need to better understand the specific pathways perturbed in DLBCL for developing effective therapeutic approaches. Mice deficient in the E3 ubiquitin ligase Smurf2 spontaneously develop B-cell lymphomas that resemble human DLBCL with molecular features of germinal centre or post-germinal centre B cells. Here we show that Smurf2 mediates ubiquitination and degradation of YY1, a key germinal centre transcription factor. Smurf2 deficiency enhances YY1-mediated transactivation of c-Myc and B-cell proliferation. Furthermore, Smurf2 expression is significantly decreased in primary human DLBCL samples, and low levels of Smurf2 expression correlate with inferior survival in DLBCL patients. The Smurf2-YY1-c-Myc regulatory axis represents a novel pathway perturbed in DLBCL that suppresses B-cell proliferation and lymphomagenesis, suggesting pharmaceutical targeting of Smurf2 as a new therapeutic paradigm for DLBCL. In response to antigen stimulation, B cells undergo extensive proliferation to form germinal centres (GCs) in secondary lymphoid organs [1] . As a consequence of cell proliferation, mutagenic events may occur and target cancer-causing genes. In addition, B cells in GCs undergo distinct genetic processes to generate high-affinity antibodies, including somatic hypermutation (SHM) of the variable region of the immunoglobulin gene and class switch recombination (CSR) that changes immunoglobulin class. These processes can target non-immunoglobulin genes in the GC B cells, leading to genetic alterations that promote tumourigenesis [2] , [3] , [4] , [5] , [6] , [7] , [8] . To counteract these oncogenic effects, it has been postulated that tumour suppressors function to constrain the proliferation and survival of the GC B cells that are at risk of malignant transformation. Identification of these specific tumour suppressors is critical to our understanding of malignancies that originated in the GCs. Most non-Hodgkin’s lymphomas are derived from GC B cells or B cells that have passed through the GCs [9] , [10] . Diffuse large B-cell lymphoma (DLBCL) is the most common subtype of non-Hodgkin’s lymphoma, accounting for 30–40% of all new diagnoses [11] . Significant progress has been made in our understanding of the dysregulated pathways and genetic abnormalities that govern the development of DLBCL [10] , [12] , [13] . Current chemotherapy regimens using the combination of cyclophosphamide, doxorubicin, vincristine and prednisone (CHOP), together with the anti-CD20 monoclonal antibody rituximab (R-CHOP), result in long-term remission in ~50% of DLBCL patients [14] . However, a significant fraction of DLBCL are still incurable, indicating that further understanding of the pathogenesis of this disease is needed to develop specific and effective therapeutic approaches. Recently, it has been shown that mice deficient in Smurf2 (Smad ubiquitination regulatory factor-2) spontaneously develop tumours, including lymphomas of B-cell origin, indicating that Smurf2 functions as a tumour suppressor [15] , [16] . It has been proposed that Smurf2 exerts its tumour suppressor function through its ability to maintain genomic integrity [15] and regulate senescence [16] . In this report, we find that B-cell lymphomas developed in Smurf2-deficient mice resemble human DLBCL with molecular features of GC or post-GC B cells. We discover that Smurf2 ubiquitinates YY1, a master regulator of GC transcriptional programme [17] , through which Smurf2 suppresses cell proliferation and c-Myc expression. This Smurf2-YY1-cMyc regulatory axis provides novel insight into lymphomagenesis in GC or post-GC B cells and is highly relevant in human DLBCL. B-cell lymphoma in Smurf2-deficient mice resembles DLBCL Previously, we have shown that Smurf2-deficient ( Smurf2 T/T , T for the gene-trapped Smurf2 allele) or the heterozygous Smurf2 +/T mice exhibit increased susceptibility to spontaneous tumourigenesis after 12 months of age, with the majority of tumours (72.7%) being lymphomas in the spleen with a B-cell origin (that is, B220 + ). All tumour-bearing Smurf2 T/T or Smurf2 +/T mice have enlarged spleens [16] , prompting us to characterize spleens in mice before malignancy. Compared with wild-type mice, an increase in spleen weight relative to body weight was found in 2-month-old Smurf2 T/T mice ( Fig. 1a ; 45.2% increase, P =0.021, Student’s t -test) or Smurf2 +/T mice ( Supplementary Fig. S1a ; 22.5% increase, P =0.07, Student’s t -test). This increase in spleen weight was accompanied by an increase in total splenic cells ( Fig. 1b ) and B220 + B cells ( Fig. 1c ), meanwhile the frequency of splenic B220 + B cells remained unchanged in young Smurf2 T/T compared with wild-type mice ( Fig. 1c ). Further, we analysed B-cell development in the bone marrow and spleen using flow cytometry. Between young Smurf2 T/T and wild-type mice, we found no obvious difference in the frequencies of various B-cell subpopulations in the bone marrow ( Supplementary Figs S2 and S3 ) and spleen ( Figs 1d and 2 and Supplementary Fig. S4 ), suggesting that B-cell development and differentiation are normal in Smurf2-deficient mice. 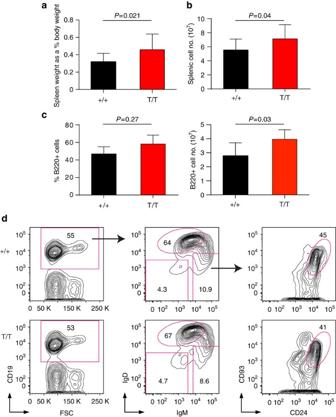Figure 1: Characterization of splenic B cells. (a) Relative gross spleen weight to body weight of 2-month-old wild-type (+/+) andSmurf2T/T(T/T) mice (N=12). (b) Total live splenic cells (N=12), and (c) per cent and total live B220+cells in spleens of 2-month-old wild-type andSmurf2T/Tmice (N=6). Error bars ina–care s.d. Student’st-test is used for statistical analysis. (d) Representative fluorescence-activated cell sorting analysis of splenic B cells from 2-month-old wild-type andSmurf2T/Tmice. Live cells (propidium iodide excluding) are displayed. The IgD++IgMintpopulation, indicated by a circular gate in the middle panel, are follicular B cells. CD93+CD24+cells, indicated by a circular gate in the right panel, are immature B cells. Frequency of each gated population as a per cent of displayed cells is shown. Figure 1: Characterization of splenic B cells. ( a ) Relative gross spleen weight to body weight of 2-month-old wild-type (+/+) and Smurf2 T/T (T/T) mice ( N =12). ( b ) Total live splenic cells ( N =12), and ( c ) per cent and total live B220 + cells in spleens of 2-month-old wild-type and Smurf2 T/T mice ( N =6). Error bars in a – c are s.d. Student’s t -test is used for statistical analysis. ( d ) Representative fluorescence-activated cell sorting analysis of splenic B cells from 2-month-old wild-type and Smurf2 T/T mice. Live cells (propidium iodide excluding) are displayed. The IgD ++ IgM int population, indicated by a circular gate in the middle panel, are follicular B cells. CD93 + CD24 + cells, indicated by a circular gate in the right panel, are immature B cells. Frequency of each gated population as a per cent of displayed cells is shown. 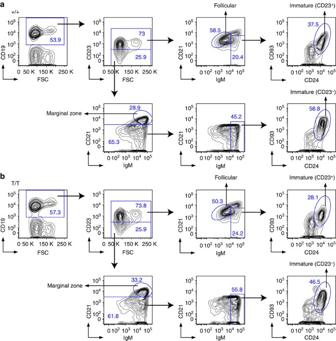Figure 2: Characterization of B cells in the spleen of Smurf2-deficient mice. Representative fluorescence-activated cell sorting analysis of splenic cells from 2-month-old (a) wild-type (+/+) and (b)Smurf2T/T(T/T) mice. Live cells (propidium iodide excluding) are displayed. Sequential gating strategies are indicated by arrows. Frequency of each gated population as a per cent of displayed cells is shown. Full size image Figure 2: Characterization of B cells in the spleen of Smurf2-deficient mice. Representative fluorescence-activated cell sorting analysis of splenic cells from 2-month-old ( a ) wild-type (+/+) and ( b ) Smurf2 T/T (T/T) mice. Live cells (propidium iodide excluding) are displayed. Sequential gating strategies are indicated by arrows. Frequency of each gated population as a per cent of displayed cells is shown. Full size image In lymphoma-bearing spleens of Smurf2-deficient mice, we observed a significant expansion (average 6.3-fold increase compared with wild-type mice) of IgD neg IgM low B cells that were CD23 negative and heterogeneous for CD24 ( Fig. 3a ), suggesting a GC or post-GC phenotype. This expansion of IgD neg IgM low B cells in tumour-bearing mice is in sharp contrast with young mice before malignancy, in which the frequency of the IgD neg IgM low B-cell population was similar between young Smurf2-deficient and wild-type mice ( Fig. 1d ). Consistent with being GC derived, these lymphomas showed positive staining for the GC markers peanut agglutinin and CD95 ( Fig. 3b,c ), underwent CSR to immunoglobulin γ2a ( Fig. 3c and Supplementary Fig. S5 ) and exhibited increased SHM in the immunoglobulin heavy chain ( IgH ) locus ( Supplementary Table S1 ). Moreover, these lymphomas showed a gene expression pattern analogous to that in human DLBCL ( Supplementary Fig. S6a ). Collectively, these data indicate that lymphomas developed in Smurf2-deficient mice are GC or post-GC derived and have molecular features consistent with DLBCL [18] . 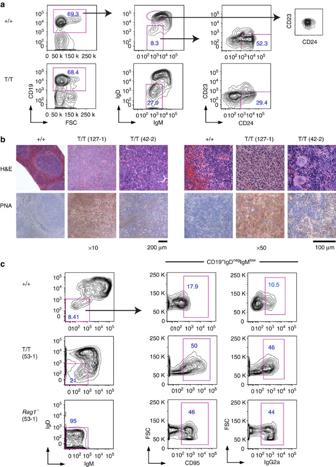Figure 3: Characterization of B-cell lymphomas generated in Smurf2-deficient mice. (a) Representative fluorescence-activated cell sorting (FACS) analysis of splenic cells from lymphoma-bearingSmurf2T/T(T/T) and age-matched wild-type (+/+) mice. Frequency of each gated population as a per cent of displayed cells is shown. CD23−CD24+cells in the right panel are activated or previously activated B cells. The CD23 versus CD24 plot for follicular B cells (IgD++IgMint) in wild-type mice is provided for comparison. (b) Representative haematoxylin and eosin and peanut agglutinin staining of lymphomas in spleen ofSmurf2T/Tmice and wild-type mouse spleen. Scale bars, 200 μm ( × 10) and 100 μm ( × 50). (c) Representative FACS analysis of CD19+splenic B cells from a lymphoma-bearingSmurf2T/Tmouse and aRag1−/−recipient mouse injected with spleen cells from this lymphoma-bearing mouse are presented. An age-matched wild-type mouse is analysed as a control, and CD19+IgDnegIgMlowpopulation gated for CD95 or IgG2a is shown for comparison. Mice used in these studies were between 15 and 18 months of age. Figure 3: Characterization of B-cell lymphomas generated in Smurf2-deficient mice. ( a ) Representative fluorescence-activated cell sorting (FACS) analysis of splenic cells from lymphoma-bearing Smurf2 T/T (T/T) and age-matched wild-type (+/+) mice. Frequency of each gated population as a per cent of displayed cells is shown. CD23 − CD24 + cells in the right panel are activated or previously activated B cells. The CD23 versus CD24 plot for follicular B cells (IgD ++ IgM int ) in wild-type mice is provided for comparison. ( b ) Representative haematoxylin and eosin and peanut agglutinin staining of lymphomas in spleen of Smurf2 T/T mice and wild-type mouse spleen. Scale bars, 200 μm ( × 10) and 100 μm ( × 50). ( c ) Representative FACS analysis of CD19 + splenic B cells from a lymphoma-bearing Smurf2 T/T mouse and a Rag1 −/− recipient mouse injected with spleen cells from this lymphoma-bearing mouse are presented. An age-matched wild-type mouse is analysed as a control, and CD19 + IgD neg IgM low population gated for CD95 or IgG2a is shown for comparison. Mice used in these studies were between 15 and 18 months of age. Full size image We analysed the genomic rearrangements of the IgH locus in representative lymphoma-bearing spleen samples and detected a specific V(D)J rearrangement in some lymphoma samples ( Supplementary Fig. S6b ), consistent with a clonal origin of these lymphomas. The lack of detection of a rearrangement using the largest V H family (J588) in other lymphoma samples may reflect the presence of non-neoplastic cells in spleen samples, rearrangement with a different V H family, or oligoclonal origin. To further investigate tumorigenicity of Smurf2-deficient lymphomas, we injected splenic cells from lymphoma-bearing Smurf2-deficient mice into sublethally irradiated Rag1 knockout ( Rag1 −/− ) mice. Rag1 −/− recipient mice became moribund 6–8 weeks after injection. An extensive expansion of IgD neg IgM low B cells was observed in the spleens of these Rag1 −/− recipients ( Fig. 3c ). Although injected splenic cells contained 1.2–1.3 × 10 5 IgD neg IgM low B cells, 1.7–8.2 × 10 6 IgD neg IgM low B cells were recovered in Rag1 −/− mice, representing a 13- to 67-fold increase of this population. Furthermore, these IgD neg IgM low B cells stained positively for CD95, consistent with a GC-derived phenotype ( Fig. 3c ). Positive staining for IgG2a confirmed that these tumours underwent CSR ( Fig. 3c ). Given that the expanded population of IgD neg IgM low B cells in Rag1 −/− mice had the same GC B-cell phenotype as the injected tumour cells, and that the recipient Rag1 −/− mice became moribund, these data are consistent with transfer of disease resembling DLBCL. Enhanced proliferation in Smurf2-deficient splenic B cells Lymphomas found in Smurf2-deficient mice showed an increase in the frequency of cells positive for the cell proliferation-associated antigen Ki-67 compared with spleen sections of age-matched wild-type mice ( Fig. 4a ). Interestingly, Ki-67 staining was increased in the spleen, particularly the white pulp, of 2-month-old Smurf2 T/T ( Fig. 4b,c ) or Smurf2 +/T mice ( Supplementary Fig. S1b ) compared with wild-type littermates. Furthermore, increased bromodeoxyuridine (BrdU) incorporation was detected in B220 + splenic B cells ( Fig. 4d ) or total splenic cells ( Supplementary Fig. S7a ) of young Smurf2 T/T mice compared with wild-type littermates. Taken together, these results suggest that increased cell proliferation observed in Smurf2-deficient splenic B cells and B-cell lymphomas is caused by reduced Smurf2 expression rather than as a consequence of tumourigenesis. 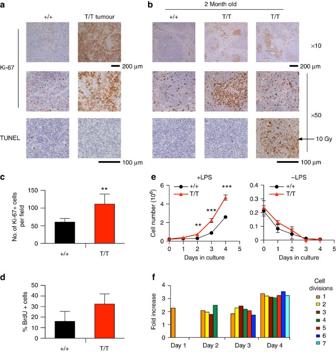Figure 4: Enhanced proliferation of splenic B cells in Smurf2-deficient mice. (a) Representative Ki-67 and TUNEL staining of lymphomas inSmurf2T/T(T/T) mice. Staining of spleen sections of aged wild-type (+/+) mice is shown for comparison. (b) Representative Ki-67 and TUNEL staining of spleen sections of 2-month-old wild-type andSmurf2T/Tmice. TUNEL staining of spleen sections of an irradiated (10 Gy) mouse is shown for comparison. Scale bars, 200 μm ( × 10) and 100 μm ( × 50). (c) Quantitation of Ki-67-positive cells in ten randomly selected fields in spleen sections of 2-month-old wild-type andSmurf2T/Tmice. (d) Analysis of BrdU incorporation in B220+splenic cells of 2-month-old wild-type andSmurf2T/Tmice (N=3). (e) Splenic cells from 2-month-old wild-type andSmurf2T/Tmice are cultured with or without LPS. The number of B220+viable cells (propidium iodide-negative) is determined by flow cytometry. Average of three independent experiments is shown. (f) The number of B220+cells undergoing different numbers of cell division is determined by CFSE staining and flow cytometry. The ratio of the number of B220+Smurf2T/Tcells undergoing different cell divisions over that of wild-type cells in one representative experiment is presented. Error bars inc–eare s.d. of at least three independent experiments. Student’st-test is used to compareSmurf2T/Tsamples with wild-type samples. **P<0.01 and ***P<0.001. Figure 4: Enhanced proliferation of splenic B cells in Smurf2-deficient mice. ( a ) Representative Ki-67 and TUNEL staining of lymphomas in Smurf2 T/T (T/T) mice. Staining of spleen sections of aged wild-type (+/+) mice is shown for comparison. ( b ) Representative Ki-67 and TUNEL staining of spleen sections of 2-month-old wild-type and Smurf2 T/T mice. TUNEL staining of spleen sections of an irradiated (10 Gy) mouse is shown for comparison. Scale bars, 200 μm ( × 10) and 100 μm ( × 50). ( c ) Quantitation of Ki-67-positive cells in ten randomly selected fields in spleen sections of 2-month-old wild-type and Smurf2 T/T mice. ( d ) Analysis of BrdU incorporation in B220 + splenic cells of 2-month-old wild-type and Smurf2 T/T mice ( N =3). ( e ) Splenic cells from 2-month-old wild-type and Smurf2 T/T mice are cultured with or without LPS. The number of B220 + viable cells (propidium iodide-negative) is determined by flow cytometry. Average of three independent experiments is shown. ( f ) The number of B220 + cells undergoing different numbers of cell division is determined by CFSE staining and flow cytometry. The ratio of the number of B220 + Smurf2 T/T cells undergoing different cell divisions over that of wild-type cells in one representative experiment is presented. Error bars in c – e are s.d. of at least three independent experiments. Student’s t -test is used to compare Smurf2 T/T samples with wild-type samples. ** P <0.01 and *** P <0.001. Full size image To further analyse cell proliferation in splenic B cells, we cultured total spleen cells of 2-month-old wild-type or Smurf2 T/T mice with the B-cell mitogen lipopolysaccharide (LPS). In response to LPS, Smurf2 T/T splenic B220 + B cells proliferated significantly better than wild-type cells ( Fig. 4e ), whereas cell viability was similar between them ( Supplementary Fig. S7b ). Using carboxyfluorescein succinimidyl ester (CFSE) to track cell divisions in cultured splenic B cells, we found that the number of Smurf2 T/T splenic B cells undergoing successive cell divisions was significantly increased compared with that of wild-type cells ( Fig. 4f and Supplementary Fig. S7c ). Without LPS stimulation, cell death was similar between wild-type and Smurf2 T/T B cells ( Fig. 4e and Supplementary Fig. S7b ). Furthermore, TUNEL (terminal deoxynucleotidyl transferase dUTP nick end labelling) staining for apoptosis was similar when spleen sections from 2-month-old Smurf2 T/T mice or lymphomas were compared with age-matched wild-type mice ( Fig. 4a,b ). Both observations suggest that apoptosis is unchanged in Smurf2-deficient cells. Collectively, these results indicate that cell proliferation is enhanced in Smurf2 T/T splenic B cells, suggesting a possible mechanism underlying increased B-cell lymphomagenesis in Smurf2-deficient mice. Elevated c-Myc expression in Smurf2-deficient mice As upregulation of c-Myc is frequently observed in B-cell lymphoma and forced expression of c-Myc drives lymphomagenesis in mice [19] , [20] , [21] , it prompted us to examine c-Myc expression in lymphomas derived from Smurf2 T/T or Smurf2 +/T mice. The expression of c-Myc mRNA in these lymphomas was increased compared with spleens of wild-type mice of the similar age ( Fig. 5a ), whereas no IgH-Myc translocation was detected in lymphomas in Smurf2-deficient mice ( Supplementary Fig. S8 ). 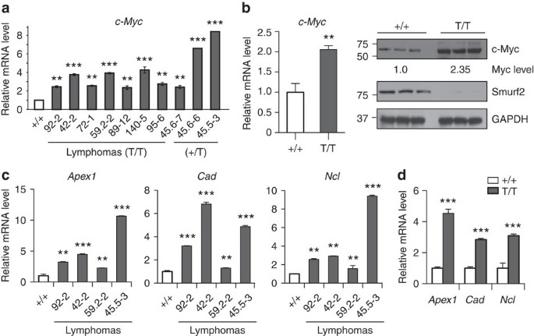Figure 5: Elevated c-Myc expression in Smurf2-deficient mice. (a) Quantitative RT–PCR analysis ofc-Mycexpression in lymphomas inSmurf2T/T(T/T) orSmurf2+/T(+/T) mice compared with spleen of aged wild-type (+/+) mice. (b) Quantitative RT–PCR and western blot analyses of c-Myc expression in spleen of 2-month-old wild-type andSmurf2T/Tmice. Larger images of immunoblots are shown inSupplementary Fig. S11a. Quantitative RT–PCR analysis of c-Myc target genes in (c) representative lymphomas fromSmurf2T/Tmice compared with spleen of aged wild-type mice and (d) spleen of 2-month-old wild-type andSmurf2T/Tmice. Error bars are s.d. of three independent experiments. Student’st-test is used to compareSmurf2T/Tsamples with wild-type samples. **P<0.01 and ***P<0.001. Figure 5: Elevated c-Myc expression in Smurf2-deficient mice. ( a ) Quantitative RT–PCR analysis of c-Myc expression in lymphomas in Smurf2 T/T (T/T) or Smurf2 +/T (+/T) mice compared with spleen of aged wild-type (+/+) mice. ( b ) Quantitative RT–PCR and western blot analyses of c-Myc expression in spleen of 2-month-old wild-type and Smurf2 T/T mice. Larger images of immunoblots are shown in Supplementary Fig. S11a . Quantitative RT–PCR analysis of c-Myc target genes in ( c ) representative lymphomas from Smurf2 T/T mice compared with spleen of aged wild-type mice and ( d ) spleen of 2-month-old wild-type and Smurf2 T/T mice. Error bars are s.d. of three independent experiments. Student’s t -test is used to compare Smurf2 T/T samples with wild-type samples. ** P <0.01 and *** P <0.001. Full size image To understand whether c-Myc elevation underlies increased B-cell proliferation and lymphomagenesis in Smurf2-deficient mice, we examined c-Myc expression in young Smurf2 T/T mice at the pre-neoplastic stage. We found an increase in c-Myc expression in the spleen ( Fig. 5b ) and liver ( Supplementary Fig. S9a,b ) of 2-month-old Smurf2 T/T mice compared with age-matched wild-type mice, suggesting that Smurf2 deficiency leads to increased c-Myc expression. To further corroborate c-Myc mRNA elevation with Smurf2 deficiency, we examined the transcript levels of c-Myc transactivation targets Apex1 , Cad and Ncl , which have been validated as c-Myc targets in multiple studies, but are not directly involved in cell proliferation ( http://www.myccancergene.org/site/mycTargetDB.asp ) [22] . We found increased transcript levels of these c-Myc targets in lymphomas ( Fig. 5c ), as well as the spleen ( Fig. 5d ) and liver of young Smurf2 T/T mice ( Supplementary Fig. S9c ). Smurf2 ubiquitinates YY1 to regulate c-Myc expression To investigate the underlying mechanism of Smurf2-mediated regulation of c-Myc expression, we searched for transcriptional regulators that have been shown to transactivate c-Myc and examined their potential as the ubiquitination targets of Smurf2. We reasoned that stabilization of such a transcriptional regulator in Smurf2-deficient mice could be responsible for elevated expression of c-Myc . YY1, which transactivates c-Myc [23] , [24] and is a central regulator of the GC B-cell-specific transcriptional programme [17] , contains a PPDY motif that can potentially interact with the WW domains in Smurf2. We found that the protein levels of YY1 were increased in lymphomas derived from Smurf2 T/T or Smurf2 +/T mice ( Fig. 6a ), as well as in the spleen ( Fig. 6b ) and liver ( Supplementary Fig. S9b ) of young Smurf2 T/T mice compared with wild-type littermates. In contrast, the transcript level of YY1 was largely unchanged in Smurf2-deficient mice ( Fig. 6b ), suggesting a post-transcriptional regulation of YY1 by Smurf2. Supporting this notion, the protein half-life of YY1 was increased from 2.1-h in wild-type splenic B cells to 4.4-h in splenic B cells of Smurf2 T/T mice ( Fig. 6c ), suggesting that Smurf2 deficiency leads to an increase in protein stability of YY1. 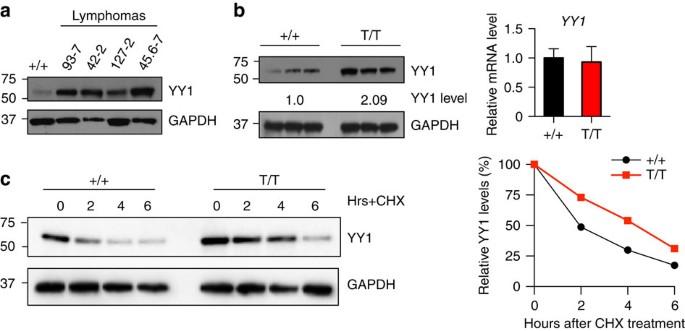Figure 6: Smurf2 regulates the stability of YY1 protein. (a) Western analysis of YY1 expression in lymphomas compared with spleen of aged wild-type (+/+) mice. (b) Western and quantitative RT–PCR analyses of YY1 expression in spleens of 2-month-old wild-type andSmurf2T/T(T/T) mice. Error bars are s.d. of three independent experiments. (c) Stability of YY1 protein is determined in splenic B cells from 2-month-old wild-type andSmurf2T/Tmice after treatment with cycloheximide (CHX). The levels of YY1 protein at time 0 are set as 100%. Larger images of immunoblots are shown inSupplementary Fig. S11b. Figure 6: Smurf2 regulates the stability of YY1 protein. ( a ) Western analysis of YY1 expression in lymphomas compared with spleen of aged wild-type (+/+) mice. ( b ) Western and quantitative RT–PCR analyses of YY1 expression in spleens of 2-month-old wild-type and Smurf2 T/T (T/T) mice. Error bars are s.d. of three independent experiments. ( c ) Stability of YY1 protein is determined in splenic B cells from 2-month-old wild-type and Smurf2 T/T mice after treatment with cycloheximide (CHX). The levels of YY1 protein at time 0 are set as 100%. Larger images of immunoblots are shown in Supplementary Fig. S11b . Full size image To further characterize Smurf2-mediated regulation of YY1, we stably expressed short-hairpin RNA (shRNA) targeting Smurf2 in a human DLBCL cell line (SUDHL-6), and found that downregulation of Smurf2 led to an increase in YY1 protein ( Fig. 7a ). Conversely, ectopic expression of Smurf2 resulted in a reduction in the steady-state level of YY1 protein. In contrast, a ligase mutant C716A, in which the conserved cysteine at residue 716 is replaced by alanine to abolish its E3 ubiquitin ligase activity [25] , [26] , [27] , did not lead to changes in YY1 ( Fig. 7b ), indicating that the regulation of YY1 by Smurf2 requires its ubiquitin ligase activity. Consistent with what we found in Smurf2-deficient mice ( Fig. 5 ), c-Myc transcripts were regulated by Smurf2 ( Fig. 7a,b ). In contrast, YY1 transcripts were largely unchanged when Smurf2 expression was altered ( Fig. 7a,b ), consistent with the notion that Smurf2 regulates YY1 post-transcriptionally. These results led us to hypothesize that Smurf2 is the E3 ubiquitin ligase responsible for ubiquitination of YY1. 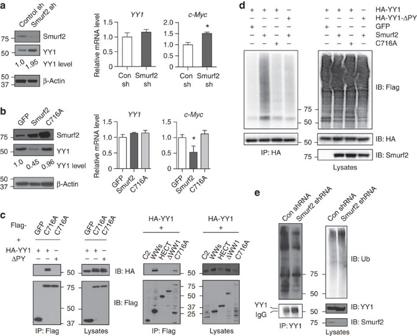Figure 7: Smurf2 mediates ubiquitination of YY1. (a) Smurf2 expression is knocked down by shRNA, and (b) Smurf2 or ligase mutant C716A is ectopically expressed in human DLBCL cells SUDHL-6. The expression of YY1 or c-Myc is analysed in western blott and quantitative RT–PCR analyses. Error bars are s.d. of three independent experiments. Student’st-test is used for statistical analysis. *P<0.05. (c) Smurf2 interacts with YY1. 293T cells are transfected with indicated constructs, and immunoprecipitation (IP) with anti-Flag antibody is followed by immunoblotting (IB) with anti-HA antibody. Larger images of immunoblots are shown inSupplementary Figs S11c and S12. (d) Smurf2 ubiquitinates YY1. 293T cells are transfected with HA-YY1 (or ΔPY), 3xFlag-Ub and Smurf2 (or C716A). IP with anti-HA antibody is followed by IB with anti-Flag antibody to detect polyubiquitinated YY1. (e) Downregulation of Smurf2 by shRNA results in decreased ubiquitination of endogenous YY1 in human DLBCL cell line SUDHL-6. IP with anti-YY1 antibody is followed by IB with anti-ubiquitin antibody to detect polyubiquitinated YY1. Larger images of immunoblots are shown inSupplementary Fig. S13a. Figure 7: Smurf2 mediates ubiquitination of YY1. ( a ) Smurf2 expression is knocked down by shRNA, and ( b ) Smurf2 or ligase mutant C716A is ectopically expressed in human DLBCL cells SUDHL-6. The expression of YY1 or c-Myc is analysed in western blott and quantitative RT–PCR analyses. Error bars are s.d. of three independent experiments. Student’s t -test is used for statistical analysis. * P <0.05. ( c ) Smurf2 interacts with YY1. 293T cells are transfected with indicated constructs, and immunoprecipitation (IP) with anti-Flag antibody is followed by immunoblotting (IB) with anti-HA antibody. Larger images of immunoblots are shown in Supplementary Figs S11c and S12 . ( d ) Smurf2 ubiquitinates YY1. 293T cells are transfected with HA-YY1 (or ΔPY), 3xFlag-Ub and Smurf2 (or C716A). IP with anti-HA antibody is followed by IB with anti-Flag antibody to detect polyubiquitinated YY1. ( e ) Downregulation of Smurf2 by shRNA results in decreased ubiquitination of endogenous YY1 in human DLBCL cell line SUDHL-6. IP with anti-YY1 antibody is followed by IB with anti-ubiquitin antibody to detect polyubiquitinated YY1. Larger images of immunoblots are shown in Supplementary Fig. S13a . Full size image To test this hypothesis, we first investigated whether Smurf2 interacts with YY1, as the C2-WW-HECT class of E3 ligases interacts with their protein substrates to catalyse ubiquitination. To limit potential degradation of YY1 by Smurf2, we used the ligase mutant C716A in co-immunoprecipitation with YY1. Smurf2 and YY1 were found to form a complex by co-immunoprecipitation, whereas deletion of the PPDY motif of YY1 (ΔPY) abolished the Smurf2-YY1 interaction ( Fig. 7c ). Furthermore, we found that three WW domains (that is, WWs), but not the C2 or HECT domain of Smurf2 alone, were sufficient to interact with YY1. Deletion of the amino terminal WW domain (ΔWW1) abolished the interaction between Smurf2 and YY1 ( Fig. 7c ). Collectively, these results indicate that the Smurf2–YY1 interaction is mediated by the WW domains of Smurf2 and the PPDY motif of YY1. We next investigated whether Smurf2 induces ubiquitination of YY1. Ubiquitination of YY1 was greatly induced in the presence of Smurf2 compared with a green fluorescent protein (GFP) control, whereas catalytically inactive C716A lost the ability to ubiquitinate YY1 ( Fig. 7d and Supplementary Fig. S10 ). Furthermore, deletion of the PPDY motif in YY1 diminished Smurf2-mediated ubiquitination ( Fig. 7d and Supplementary Fig. S10 ). Conversely, we used stably expressed shRNA to knock down the expression of Smurf2 in SUDHL-6 cells, and found that downregulation of Smurf2 resulted in decreased ubiquitination of endogenous YY1 ( Fig. 7e ). Collectively, these results indicate that Smurf2 is the E3 ubiquitin ligase responsible for ubiquitination of YY1. YY1 has been shown to bind to the human c-Myc promoter in a chromatin immunoprecipitation (ChIP) assay and to be sufficient to upregulate c-Myc expression [23] , [24] . We expressed shRNA to knockdown YY1 expression in SUDHL-6 cells, and found that c-Myc transcripts were decreased upon YY1 downregulation ( Fig. 8a ), indicating that YY1 is required to regulate c-Myc expression. As shRNA knockdown of Smurf2 expression in SUDHL-6 cells led to elevation of c-Myc, further downregulation of YY1 by shRNA resulted in decreased c-Myc expression ( Fig. 8b ), suggesting that YY1 is the critical mediator of Smurf2-regulated c-Myc expression. Further supporting this notion, knockdown of YY1 expression by siRNA led to downregulation of c-Myc in primary B cells isolated from spleens of wild-type and Smurf2 T/T mice ( Fig. 8c ). Moreover, ChIP analysis indicated that YY1 was bound to the c-Myc promoter in mouse spleen, and this binding was increased in spleen of Smurf2 T/T mice compared with wild-type mice ( Fig. 8d ), consistent with the mechanism in which stabilization of YY1 in Smurf2-deficient cells upregulates c-Myc expression. 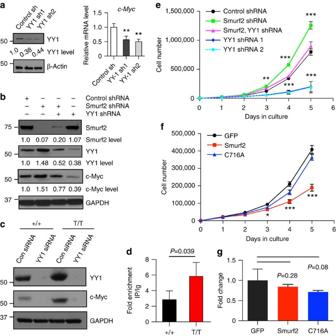Figure 8: Smurf2-YY1 regulates c-Myc expression and cell proliferation. (a) Downregulation of YY1 by shRNA (left image) leads to decreased c-Myc in human DLBCL cell line SUDHL-6 as determined by quantitative RT–PCR (right image). (b) Western blot analysis of c-Myc expression in SUDHL-6 cells after shRNA-mediated knockdown ofSmurf2orYY1expression. (c) Knockdown ofYY1by siRNA leads to downregulation of c-Myc in splenic B cells of wild-type (+/+) andSmurf2T/T(T/T) mice. (d) ChIP assay of YY1 binding onto thec-Mycpromoter in spleens of 2-month-old wild-type andSmurf2T/Tmice. Fold enrichment of ChIP with anti-YY1 antibody over IgG control is shown. (e) Growth curves of human DLBCL cell line SUDHL-6 after shRNA-mediated knockdown ofSmurf2orYY1expression. (f) Growth curves and (g) apoptosis assay of SUDHL-6 cells after ectopic expression of Smurf2, ligase mutant C716A or GFP control. Error bars are s.d. of three independent experiments. Cells with shRNA knockdown or Smurf2 expression were compared with control shRNA or GFP, respectively, using Student’st-test. *P<0.05, **P<0.01 and ***P<0.001. Larger images of immunoblots are shown inSupplementary Fig. S13b. Figure 8: Smurf2-YY1 regulates c-Myc expression and cell proliferation. ( a ) Downregulation of YY1 by shRNA (left image) leads to decreased c-Myc in human DLBCL cell line SUDHL-6 as determined by quantitative RT–PCR (right image). ( b ) Western blot analysis of c-Myc expression in SUDHL-6 cells after shRNA-mediated knockdown of Smurf2 or YY1 expression. ( c ) Knockdown of YY1 by siRNA leads to downregulation of c-Myc in splenic B cells of wild-type (+/+) and Smurf2 T/T (T/T) mice. ( d ) ChIP assay of YY1 binding onto the c-Myc promoter in spleens of 2-month-old wild-type and Smurf2 T/T mice. Fold enrichment of ChIP with anti-YY1 antibody over IgG control is shown. ( e ) Growth curves of human DLBCL cell line SUDHL-6 after shRNA-mediated knockdown of Smurf2 or YY1 expression. ( f ) Growth curves and ( g ) apoptosis assay of SUDHL-6 cells after ectopic expression of Smurf2, ligase mutant C716A or GFP control. Error bars are s.d. of three independent experiments. Cells with shRNA knockdown or Smurf2 expression were compared with control shRNA or GFP, respectively, using Student’s t -test. * P <0.05, ** P <0.01 and *** P <0.001. Larger images of immunoblots are shown in Supplementary Fig. S13b . Full size image Smurf2 and YY1 regulate proliferation of DLBCL cells To understand the consequence of Smurf2-mediated ubiquitination of YY1 in lymphomagenesis, we investigated the Smurf2–YY1 axis in regulation of cell proliferation in human DLBCL cells. Consistent with our observation of increased cell proliferation in Smurf2-deficient mice, shRNA knockdown of Smurf2 expression in SUDHL-6 cells ( Fig. 8b ) led to enhanced cell proliferation ( Fig. 8e ). Downregulation of YY1 by shRNA ( Fig. 8b ) resulted in decreased proliferation in SUDHL-6 cells, indicating that YY1 is a critical regulator of cell proliferation in DLBCL cells ( Fig. 8e ). Furthermore, downregulation of YY1 in SUDHL-6 cells that already had shRNA knockdown of Smurf2 ( Fig. 8b ) alleviated the increase in cell proliferation mediated by Smurf2 deficiency ( Fig. 8e ), suggesting that Smurf2 regulates cell proliferation through YY1. Conversely, ectopic expression of wild-type Smurf2, but not the ligase mutant C716A, in SUDHL-6 cells ( Fig. 7b ) led to significantly decreased cell proliferation ( Fig. 8f ), whereas apoptosis was not significantly changed ( Fig. 8g ). Taken together, these results indicate the Smurf2-YY1 regulatory axis is critical in proliferation of lymphoma cells, providing a plausible mechanism underlying increased cell proliferation and lymphomagenesis in Smurf2-deficient mice. Smurf2 expression correlates with DLBCL patient survival To investigate whether Smurf2 deficiency has clinical relevance in human lymphomagenesis, we analysed Smurf2 expression in primary human lymphoma samples. In a published microarray data set (GSE2350) that contains samples of human primary B-cell lymphoma and normal B cells [28] , we found that the expression of Smurf2 was significantly decreased in DLBCL, Burkitt’s lymphoma (BL) and follicular lymphoma compared with normal B cells ( Fig. 9a ). 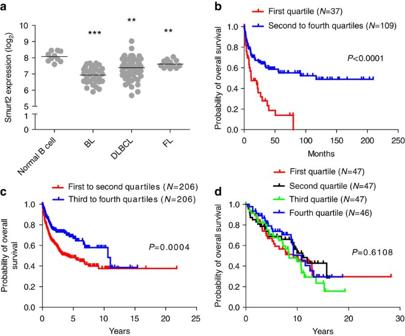Figure 9: The level of Smurf2 expression correlates with overall survival of human DLBCL patients. (a) Dot plot of Smurf2 expression in normal B cells (N=10), BL (N=33), DLBCL (N=60) and follicular lymphoma (FL,N=14). One-way analysis of variance is used to compare tumours with normal B cells. **P<0.01 and ***P<0.001. Kaplan–Meier curves of overall survival of patients in human B-cell lymphoma data sets (b) GSE4475, (c) GSE10846 and (d) an FL data set plotted according to the level of Smurf2 expression, with the first quartile having the lowest Smurf2 expression. The log-rank test is used for statistical analysis. Figure 9: The level of Smurf2 expression correlates with overall survival of human DLBCL patients. ( a ) Dot plot of Smurf2 expression in normal B cells ( N =10), BL ( N =33), DLBCL ( N =60) and follicular lymphoma (FL, N =14). One-way analysis of variance is used to compare tumours with normal B cells. ** P <0.01 and *** P <0.001. Kaplan–Meier curves of overall survival of patients in human B-cell lymphoma data sets ( b ) GSE4475, ( c ) GSE10846 and ( d ) an FL data set plotted according to the level of Smurf2 expression, with the first quartile having the lowest Smurf2 expression. The log-rank test is used for statistical analysis. Full size image To further understand the relevance of decreased Smurf2 expression in human lymphomagenesis, we next investigated whether the level of Smurf2 expression correlates with clinical outcome. Smurf2 expression has been measured in three human primary B-cell lymphoma microarray data sets, each of which contains survival information of more than 100 patients [29] , [30] , [31] . Within each data set, we divided lymphoma samples into four groups based on the level of Smurf2 expression, with the first quartile having the lowest Smurf2 expression. Survival analysis of data set GSE4475 in the Gene Expression Omnibus (GEO, http://www.ncbi.nlm.nih.gov/geo ), which contains DLBCL and some BL patients [29] , showed that overall survival of patients with the lowest Smurf2 expression (first quartile) was significantly worse ( P <0.0001, log-rank test) than that of patients with higher Smurf2 expression (second to fourth quartile; Fig. 9b ). Similarly, a significantly poor survival prognosis ( P =0.0004, log-rank test) was observed in patients with low level of Smurf2 expression (first and second quartiles) compared with patients with high level of Smurf2 expression (third and fourth quartiles) in an independent data set GSE10846 in GEO ( Fig. 9c ), which contains only DLBCL patients [30] . Interestingly, we found no significant difference in overall survival of patients in a human follicular lymphoma data set [31] based on Smurf2 expression level ( Fig. 9d ), suggesting a specific role of Smurf2 deficiency in human DLBCL or possibly BL. Certain clinical and molecular parameters have been shown to predict DLBCL patient survival [32] , [33] , [34] . Univariate analysis indicated a significant correlation between poor survival prognosis and age, Ann Arbor stage, molecular subtype or International Prognostic Index (IPI) score. To determine whether Smurf2 expression can predict clinical outcomes independently of these known parameters, we carried out a multivariate Cox regression analysis and found that low level of Smurf2 expression was an independent predictor of patient survival in both DLBCL cohorts ( P =0.01 for GSE4475 and P =0.027 for GSE10846; Table 1 ). These results indicate that Smurf2 expression is a valuable prognostic marker for DLBCL patient survival, and further suggest that Smurf2 is a potential therapeutic target for DLBCL. Table 1 Univariate and multivariate analyses of prognostic factors associated with DLBCL patient overall survival. Full size table In this study, we found that lymphomas developed in Smurf2-deficient mice have molecular features of GC or post-GC B cells and resemble human DLBCL. A significant decrease in Smurf2 expression is found in human DLBCL compared with normal B cells, indicating the clinical relevance of Smurf2 deficiency in human lymphomagenesis. Furthermore, our finding that low levels of Smurf2 expression correlate with poor survival prognosis in DLBCL patients suggests that Smurf2 is part of an important molecular pathway controlling lymphoma development. This pathway, identified in this study as the Smurf2-YY1-c-Myc regulatory axis, is novel and specific in suppression of B-cell proliferation and consequently lymphomagenesis. To our knowledge, Smurf2 is the first E3 ligase identified to ubiquitinate YY1. As a transcriptional regulator, YY1 has a critical role in many biological processes, including development, differentiation and proliferation, and has been implicated in oncogenesis [35] , [36] . Specific to B cells, YY1 is a critical regulator of B-cell development [37] and has recently been identified as a central regulator of the GC B-cell-specific transcriptional programme [17] . The expression of YY1 is found to be increased in high-grade DLBCL or BL compared with low-grade lymphoma or normal B cells [38] . Furthermore, elevated YY1 expression correlates with poor survival prognosis of DLBCL patients [39] , suggesting an oncogenic function for YY1 in human B-cell lymphomagenesis. The Smurf2-YY1-c-Myc regulatory axis is thus a useful prognostic predictor of clinical outcome in DLBCL patients and a potential therapeutic target for treatment of DLBCL. There is no evidence that the Smurf2 locus is deleted in human DLBCL [40] , [41] or BL [42] , [43] , suggesting that epigenetic regulation probably has an important role in Smurf2 deficiency in human lymphomagenesis. Moreover, we showed that restoration of Smurf2 expression in human DLBCL cells can suppress cell proliferation ( Fig. 8f ), providing an opportunity to design strategies to increase the expression of Smurf2 in lymphomas as a new therapeutic approach complementing current CHOP/R-CHOP regimens. Increased susceptibility to B-cell lymphomagenesis in Smurf2-deficient mice is preceded by enhanced proliferation in splenic B cells. B cells undergo SHM and CSR in GCs to generate high-affinity antibodies. Both SHM and CSR are mutagenic and may target non-immunoglobulin genes. These ‘off-target’ genetic alterations contribute to lymphomagenesis [2] , [3] , [4] , [5] , [6] , [7] , [8] . Enhanced proliferation would predispose Smurf2-deficient B cells to these mutagenic events, which ultimately contribute to lymphomagenesis. Consistent with this notion, Smurf2-deficient mice develop lymphomas at 12–15 months of age, most probably reflecting the infrequent generation of splenic GCs in un-immunized mice along with the accumulation of mutations with age. Recently, it has been shown that Smurf2 regulates histone H2B monoubiquitination by targeting the ring finger protein 20 for ubiquitination and degradation. Loss of Smurf2 leads to genomic instability through alterations in histone modification [15] , suggesting an important mechanism through which Smurf2 functions as a tumour suppressor. Our work now adds a novel dimension to the tumour suppressive functions of Smurf2. As YY1 has been shown to transactivate c-Myc expression [23] , [24] , our discovery of Smurf2-mediated ubiquitination and degradation of YY1 provides a novel mechanism by which Smurf2 regulates c-Myc expression and cell proliferation. Myc translocation is not common in DLBCL (5–10%); however, increased Myc expression is observed in ~30% of DLBCL and correlates with poor survival prognosis in DLBCL patients [44] . Although no IgH-Myc translocation was found, lymphomas derived from Smurf2-deficient mice all showed increased expression of c-Myc . The Smurf2-YY1-c-Myc axis identified in the present study provides a plausible mechanism for increased Myc expression without chromosomal translocation in DLBCL. As a master regulator of cell proliferation [45] , the oncogenic function of c-Myc in B-cell lymphomagenesis is well documented [19] , [20] , [21] , [46] . In response to activated oncogenes, intrinsic tumour suppression mechanisms such as apoptosis and senescence are triggered to restrain oncogenic proliferation. With c-Myc, an additional layer of complexity is provided by the exquisite sensitivity of cells to different levels of c-Myc overexpression. High level of c-Myc overexpression increases cell proliferation and drives lymphomagenesis, but also induces apoptosis [20] , [21] , [47] . Suppression of apoptosis exacerbates c-Myc-induced lymphomagenesis, suggesting that apoptosis antagonizes c-Myc’s oncogenic activity [21] . Further, it has been recently found that low level of c-Myc elevation promotes cell proliferation without inducing apoptosis [48] . Consistent with this observation, we found that Smurf2-deficient mice showed low level (~2-fold) of c-Myc elevation ( Fig. 5b ) and enhanced proliferation in B cells without significant induction of apoptosis ( Fig. 4 and Supplementary Fig. S7 ). In the absence of apoptosis, senescence is likely to become the critical tumour suppression mechanism to antagonize the oncogenic activity of Myc. A recent study shows that constitutive activation of c-Myc indeed activates senescence [49] . Smurf2 is an important regulator of senescence [16] , [50] , [51] , [52] . In Smurf2-deficient cells, impaired senescence response leads to prolonged cell proliferation, including in splenic cells [16] , suggesting that enhanced cell proliferation induced by low level of c-Myc activation coupled with an impaired senescence response drives lymphomagenesis in Smurf2-deficient mice. Smurf2 thus has multiple roles in tumour suppression by maintaining chromatin landscape and genomic stability, suppressing cell proliferation and regulating the senescence response. Smurf2-deficient mice Smurf2-deficient mice as described previously [16] have been backcrossed to C57BL/6 for >10 generations. Tissues were collected for DNA, RNA and protein preparation, or fixed in 10% phosphate-buffered formalin. Five-micrometre paraffin sections were stained for haematoxylin and eosin, and peanut agglutinin (Vector Labs), TUNEL (Roche), B220 and Ki-67 (antibody sources and dilutions in Supplementary Table S2 ). For transplantation, 2 × 10 6 splenic cells from tumour-bearing mice were injected retro-orbitally into sublethally irradiated (3 Gy) Rag1 −/− mice (Jackson Laboratories). All studies were carried out according to guidelines approved by the Institutional Animal Care and Use Committee of University of Massachusetts Medical School. Flow cytometry Spleens were collected from 2-month-old mice of both sexes and ground between frosted glass slides. Bone marrow cells were collected from long leg bones. After red blood cells were lysed, cells were filtered through a 70-μm nylon mesh and incubated with anti-CD16/32 antibody (10 min on ice). Cells were incubated with primary antibodies for 20 min and washed three times with staining media (biotin-, flavin- and phenol red-deficient RPMI-1640 medium with 10 mM, pH 7.2, HEPES, 0.02% sodium azide, 1 mM EDTA and 2% fetal bovine serum (FBS)). Antibodies (sources and dilutions in Supplementary Table S3 ) included B220-APC (RA3-6B2), CD19-PE-TR (ID3), CD21-FITC (7G6), CD23-biotin (B3B4), CD24-FITC (30-F1), CD43-PE (S7), CD93-PE-Cy7 (AA4.1), CD95-PE (15A7), CD117(c-kit)-PE-Cy5.5 (2B8), CD127-PE (A7R34), IgD-PE or -biotin (11–26), IgM-APC, -biotin or -PE-Cy7 (II/41), IgG2a-PE (m2a-15F8) and Ly6C-FITC (AL21). Biotin-stained cells were incubated with streptavidin–pacific blue (Invitrogen) for 15 min on ice, washed three times and resuspended in 1 μg ml −1 propidium iodide to exclude dead cells. Flow cytometry was performed on a 5-laser, 18-detector LSR II (BD Biosciences) and data were analysed using FlowJo (Treestar). Splenic B-cell proliferation assays Mouse spleen was collected and processed as described above. Single splenic cell suspension was treated with 10 μM CFSE (Invitrogen) for 10 min at 37 °C and cultured in RPMI-1640 medium with 10% FBS, 100 μM MEM non-essential amino acids, 2 mM glutamine and 50 μM 2-mercaptoethanol (Invitrogen) in a humidified chamber containing 5% CO 2 at 37 °C. Cells were treated with 5 μM LPS (Sigma) or left untreated. Cells were stained with anti-B220-APC antibody daily for 4 days. After being washed and resuspended in 1 μg ml −1 propidium iodide, cells were analysed by flow cytometry with BD FACSCaliber and FlowJo. Mice were injected with 1 mg BrdU (BD Biosciences) intraperitoneally. Spleen was collected 24 h later and processed as described above. Splenic cells were fixed and stained with anti-BrdU-FITC antibody using BrdU flow kit (BD Biosciences) and anti-B220-APC antibody. Data were collected by flow cytometry on BD FACSCaliber and analysed using FlowJo. Cycloheximide treatment Mouse splenic cells were collected and cultured as described above. Cells were treated with 15 μg ml −1 cycloheximide (Sigma) and cell lysates were collected every 2 h post treatment. CSR and SHM assays Transcripts of mouse IgH were amplified by quantitative reverse transcriptase (RT)–PCR as described [53] . Briefly, μ (IgM)-transcripts were amplified using primers ImF and CmR. Post-switch transcripts were amplified using the following primers: ImF and Cg1R for γ1 (IgG1), ImF and Cg2aR for γ2a (IgG2a), ImF and Cg2bR for γ2b (IgG2b), and ImF and Cg3R for γ3 (IgG3). Primers used are ImF: 5′-CTCTGGCCCTGCTTATTGTTG-3′; CmR: 5′-GAAGACATTTGGGAAGGACTGACT-3′; Cg1R: 5′-GGATCCAGAGTTCCAGGTCACT-3′; Cg2aR: 5′- GCCACATTGCAGGTGATGGA-3′; Cg2bR: 5′-CACTGAGCTGCTCATAGTGTAGAGTC-3′; and Cg3R: 5′-CTCAGGGAAGTAGCCTTTGACA-3′. The frequency of somatic mutation in mouse IgH was determined as described [53] . Briefly, V H 186.2 transcripts of mouse IgH μ-isotype were amplified in RT–PCR using Phusion hot start high-fidelity Taq Polymerase (New England Biolabs) with primers V H 186.2 (5′-TTCTTGGCAGCAACAGCTACA-3′) and CmR (5′-GAAGACATTTGGGAAGGACTGACT-3′). PCR products were cloned into pGEM-T-easy vector (Promega) and individual colonies were sequenced. Clonal analysis of mouse B-cell lymphomas Rearrangements of the variable region of mouse IgH were analysed as described [54] . Briefly, genomic DNA was prepared from lymphoma-bearing spleen of Smurf2-deficient mice or spleen of wild-type mice using classic genomic DNA isolation kit (Lamda Biotech) and used in PCR with primers V H (J558FR3: 5′-CAGCCTGACATCTGAGGACTCTGC-3′) and 3′ of J H4 (JH4int: 5′-CTCCACCAGACCTCTCTAGACAGC-3′). Analysis of IgH-Myc translocation IgH-Myc translocation in mouse B-cell lymphomas was detected as described [55] . Briefly, genomic DNA isolated from lymphomas was used as template in nested PCR using expended long PCR system (Roche). Primers were: 5′-TGAGGACCAGAGAGGGATAAAAGAGAA-3′ and 5′-GGGGAGGGGGTGTCAAATAATAAGA-3′ (first round); and 5′-CACCCTGCTATTTCCTTGTTGCTAC-3′ and 5′-GACACCTCCCTTCTACACTCTAAACCG-3′ (second round). Myc locus was amplified as controls with primers of 5′-GGGGAGGGGGTGTCAAATAATAAGA-3′ and 5′-GTGAAAACCGACTGTGGCCCTGGAA-3′. Two lymphoma samples (318 and 334) with IgH-Myc translocation [56] were kindly provided by Dr John Manis (Harvard Medical School) and used as positive controls. Cell culture and transfection SUDHL-6 cells (kindly provided by Dr. Subbarao Bondada, University of Kentucky) were cultured in RPMI-1640 medium with 10% FBS in a humidified chamber containing 5% CO 2 at 37 °C. Lentiviral vectors pLenti-CMV-Smurf2-IRES-Puro, pLenti-CMV-C716A-IRES-Puro or pLenti-CMV-GFP-IRES-Puro were described previously [51] . Briefly, fragments of Smurf2 or GFP complementary DNA were inserted into a lentiviral vector to express Smurf2 or GFP under the control of a cytomegalovirus (CMV) promoter. Lentiviral shRNA constructs targeting Smurf2 (V2LHS_10399), YY1 (V2LHS_219592, V2LHS_389741) and a non-silencing shRNA control (RHS4346) were purchased from Open Biosystems. Lentiviral packaging and infection were carried out as described [51] . Briefly, lentiviral vectors were cotransfected with a plasmid (pMD2.VSV-G) encoding vesicular stomatitis virus glycoprotein (VSV-G) and a plasmid (pCMVdR8.74) encoding packaging proteins into 293T cells. VSV-G-pseudotyped virus were collected 48 h after transfection and were used to infect target cells in the presence of 4 μg ml −1 polybrene (Sigma). Cells were fluorescence-activated cell sorted for GFP+ cells (shRNA knockdown) or selected with puromycin (1 μg ml −1 , Sigma) for 1 week. To analyse cell proliferation, sorted or selected cells were seeded at 5 × 10 3 per well in six-well plates, collected in triplicate and counted daily for 5 days using Z1 Coulter Particle Counter (Beckman Coulter). Apoptosis was measured using Caspase-Glo 3/7 assay (Promega). Splenic B cells were isolated using anti-B220-biotin antibody and anti-biotin beads with AutoMACS Pro (Miltenyi Biotec) and cultured with 5 μM LPS as described above. Cells (3 × 10 6 ) were transfected with 10 pmol YY1 siRNA (sc-36864) or control siRNA (sc-37007, Santa Cruz Biotechnology) using mouse B cell Nucleofector kit on Nucelofector I device (Lonza) with the programme Z-01. Cell lysates were collected 48 h after transfection. Quantitative RT–PCR Total RNA was isolated using RNeasy Mini kit (Qiagen) and reverse-transcribed using Superscript II (Invitrogen). Real-time PCR was performed using SYBR Green PCR kit (Bio-Rad). The following primers were used: Smurf2 (F: 5′-ATGAAGTCATTCCCCAGCAC-3′; R: 5′-AACCGTGCTCGTCTCTCTTC-3′), c-Myc (F: 5′-GGACAGTGTTCTCTGCC-3′; R: 5′-CGTCGCAGATGAAATAGG-3′), YY1 (F: 5′-TGAGAAAGCATCTGCACACC-3′; R: 5′-CGCAAATTGAAGTCCAGTGA-3′), Apex1 (F: 5′-GCTCCGTCAGACAAAGAAGG-3′; R: 5′-GCATTGGGAACATAGGCTGT-3′), Cad (F: 5′-TGGTCAGTTCATCCTCACTCC-3′; R: 5′-TACATGCCGTTCTCAGCTTG-3′), Ncl (F: 5′-TAAGGGTGAAGGTGGCTTTG-3′; R: 5′-CCTTGTGGCTTGAAGTCTCC-3′) and β-actin (F: 5′-GCTCTTTTCCAGCCTTCCTT-3′; R: 5′-GTGCTAGGAGCCAGAGCAGT-3′). Western blot and co-immunoprecipitation analysis Total cell lysates were collected using RIPA buffer (50 mM Tris-HCl, pH 7.5, 150 mM NaCl, 1% Triton X-100, 0.1% SDS, 0.5% deoxycholic acid and 0.02% sodium azide) with freshly added complete protease inhibitors (Roche). Protein lysates (20 μg) were separated by SDS–PAGE Criterion X-gel (Bio-Rad) and transferred to nitrocellulose membranes (GE Osmonics). Immunoblots were analysed by western blotting and visualized using a western lightening chemiluminescence detection kit (Perkin Elmer). Primary antibodies were Smurf2, c-Myc, YY1, Flag, HA, ubiquitin, β-actin and GAPDH (antibody sources and dilutions in Supplementary Table S2 ). For co-immunoprecipitation, cells were lysed in NP40 lysis buffer (20 mM Tris-HCl, 150 mM NaCl, 2 nM EDTA, 1% Nonidet P-40) plus complete protease inhibitors (Roche). Lysates were incubated with anti-Flag M2 affinity gel (Sigma) overnight at 4 °C. Immunoprecipitates were washed four times with NP40 lysis buffer and analysed using western blotting with anti-HA antibody. Ubiquitination assay 293T cells were transfected with HA-YY1 (a gift of Dr Yang Shi, Harvard Medical School), 3 × Flag-ubiquitin (provided by Dr Quan Lu, Harvard School of Public Health) and Smurf2. GFP and C716A were used as controls. Cells were treated with MG132 (20 μM, Sigma) for 2 h and lysed in RIPA buffer (50 mM Tris-HCl, pH 7.5, 150 mM NaCl, 1% Triton X-100, 0.1% SDS, 0.5% deoxycholic acid and 0.02% sodium azide) plus 10 mM N -ethylmaleimide (Fisher Scientific). Cell lysates were incubated with anti-HA or anti-Flag affinity gel (Sigma) overnight at 4 °C. Immunoprecipitates were washed with RIPA buffer three times and analysed using western blotting with anti-Flag or anti-HA antibody to detect ubiquitin conjugation. To detect ubiquitination of endogenous YY1 in SUDHL-6 cells, cell lysates were incubated with anti-YY1 antibody overnight at 4 °C followed by incubation with protein A-agarose (Invitrogen). Polyubiquitinated YY1 was detected by western blotting using anti-ubiquitin antibody. ChIP assay Mouse spleen was collected and processed as described above. Single-cell suspension was cross-linked using 1% formaldehyde (Sigma) in RPMI-1640 medium (room temperature for 10 min). After neutralization with glycine (125 nM), cells were lysed in SDS lysis buffer. Chromatin was sonicated to fragments of ~500 bp, and ChIP analysis with anti-YY1 antibody or matched IgG was performed using ChromaFlash one step ChIP kit (Epigentek). After reverse of cross-linking (65 °C for 3 h), the c-Myc promoter region containing the YY1-binding site was amplified in quantitative PCR with primers: F: 5′-TCCCCAGCCTTAGAGAGACG-3′ and R: 5′-GGCTCCGGGGTGTAAACAGT-3′. Chromatin before ChIP was used as input. Gene expression and statistical analyses Microarray data (GSE2350, GSE4475 and GSE10846) were retrieved from GEO ( http://www.ncbi.nlm.nih.gov/geo ). Expression of Smurf2 (log 2 transformed) was analysed with dot plot, and one-way analysis of variance was used for statistical analysis. Kaplan–Meier survival curves were plotted using GraphPad Prism 5.0 and log-rank test was used for statistical analysis. Univariate and multivariate Cox regression analyses were used to estimate the hazard ratios and 95% confidence intervals, and statistical significance was analysed using SPSS Statistics 19 software (IBM). Human DLBCL data set GSE10846 contains samples from patients receiving CHOP or R-CHOP treatment. Revised IPI score was used to group these patients: low (0), intermediate (1 or 2) or high (3, 4 or 5) (ref. 34 ). Some IPI variables were missing in some samples. If the missing IPI variables did not change the IPI grouping of a given sample, this sample was included in the analysis. Otherwise, the sample was excluded. Data were presented as mean±s.d. Two-tailed and unpaired Student’s t -test was used for pairwise comparisons, with P <0.05 considered as statistically significant. How to cite this article: Ramkumar, C. et al. Smurf2 suppresses B-cell proliferation and lymphomagenesis by mediating ubiquitination and degradation of YY1. Nat. Commun. 4:2598 doi: 10.1038/ncomms3598 (2013).